Shp1 signalling is required to establish the long-lived bone marrow plasma cell pool Germline or B-cell-specific loss of Ptpn6 gene encoding the Shp1 protein tyrosine phosphatase leads to skewed B lymphopoiesis and systemic autoimmunity. Here, to study its role in B-cell terminal differentiation, we generated Ptpn6 f/f Aicda Cre/+ mice with Shp1 ablated only in activated B cells. We show that Ptpn6 f/f Aicda Cre/+ mice have normal B-cell development but exhibit defective class-switched primary and recalled antibody response to a T-cell-dependent antigen. Germinal centres are present but do not persist and memory B cells are not formed. Interestingly, Shp1-deficient plasma cells are generated in the spleen but do not contribute to the bone marrow long-lived pool. Plasma cells lacking Shp1 exhibit aberrant α4β1 integrin activation due to dysregulated Src- and PI3-kinase signalling and manifest attenuated migration in vitro and defective bone marrow homing when reconstituted in vivo . Interrupting α4β1–VCAM-1 interaction rectifies this defect. These data suggest that Shp1 signalling is required for the establishment of a life-long protective humoral immunity. The protein tyrosine phosphatase Shp1, encoded by Ptpn6 gene, is expressed mainly in hematopoietic cells [1] , [2] , [3] . It is known to negatively regulate multiple signal transduction pathways, including those of antigen- [4] , [5] , cytokine- [6] and chemokine-receptor [7] , FAS [8] , [9] and integrins [10] , [11] , [12] . The natural mouse mutants motheaten and motheaten viable exhibit systemic inflammation and autoimmunity [13] , [14] . In these mutants, Shp1 was perturbed in multiple cell types and it was difficult to study the precise role of Shp1 in various cell functions. The role of Shp1 in different cell types was later examined with mouse mutants bearing conditional cell-type-specific deletions of Shp1 in T cells [15] , dendritic cells [16] and neutrophils [11] , and it became apparent that this phosphatase played critical roles in the differentiation and/or activation of these cells. B-cell-specific ablation of Shp1 was achieved using CD19-Cre and the resulting mouse mutant ( Ptpn6 f/f CD19 Cre/+ ) also manifested systemic autoimmunity [17] . In Ptpn6 f/f CD19 Cre/+ mice, B-cell development was perturbed with drastic reduction of follicular B cells and preferential differentiation of CD5 + B-1 cells. These mice also had disrupted splenic architecture and therefore it was difficult to study the precise role of Shp1 in follicular B-cell activation and terminal differentiation. When naive follicular B cells encounter specific antigens, they form germinal centres (GC) with T cell help and GC B cells further differentiate into antibody-secreting cells (ASCs) and memory B cells [18] , [19] , [20] . ASCs subsequently migrate to the bone marrow to occupy survival niches and form the long-lived plasma cell (PC) pool [21] , [22] , which helps to establish an individual’s life-long immunity to an antigen [23] . Recently, it was demonstrated that Shp1 was highly expressed and activated in GC B cells and when Shp1 was inducibly ablated in the midst of an on-going immune response, GC maintenance was affected [24] . However, the role of Shp1 in PC function remains to be addressed. Once formed, ASCs migrate to the bone marrow to establish the long-lived PC pool and this is in-part regulated by integrins [21] , [22] . Deficiencies in certain integrins were known to affect humoral immune response [25] , [26] . Integrins α4β1 and αLβ2 have been shown to be highly expressed on splenic ASCs [27] , [28] , [29] , [30] . The deletion of vascular cell-adhesion molecule 1 (VCAM-1), the ligand for α4β1, leads to compromised antibody responses [31] . Shp1 has been implicated in the negative regulation of ligand-binding and downstream signalling of Integrins in various cell types [10] , [11] , [32] , [33] . Whether Shp1 is involved in the signalling of integrins on ASCs and how this would affect their bone marrow homing and the establishment of long-lived humoral immunity in vivo are also not quite well understood. To elucidate the in vivo relevance of Shp1 signalling in PC differentiation, we generated Ptpn6 f/f Aicda Cre/+ mice in which Shp1 is deleted in B cells that encounter antigen. Unlike Ptpn6 f/f CD19 Cre/+ mice that preferentially developed CD5 + B-1 cells and lacked follicular B cells, Ptpn6 f/f Aicda Cre/+ mice generate normal fractions of follicular and other B-cell subsets. When Ptpn6 f/f Aicda Cre/+ mice were challenged with antigen, GCs developed but they could not persist and memory B cells were not formed. Interestingly, Shp1-deficient ASCs were generated. However, they could not contribute to the long-lived PC pool in the bone marrow. Shp1-deficient ASC exhibited aberrant activation of α4β1 integrin that affected their migratory properties and homing to bone marrow niches. Interruption of α4β1–VCAM-1 interaction corrected this defect in immunized Ptpn6 f/f Aicda Cre/+ mice. Our data indicate that Shp1 plays an important role in the establishment of life-long humoral immunity. Generation and characterization of Ptpn6 f/f Aicda Cre/+ mice To study the role of Shp1 in B-cell terminal differentiation, we generated Ptpn6 f/f Aicda Cre/+ mice that harbour Ptpn6 genes flanked by loxP sites ( Ptpn6 f/f ) and with Cre recombinase gene targeted to one of the alleles of Aicda gene. In this mouse, Shp1 is ablated only in antigen-activated B cells, which expressed the enzyme activation-induced cytidine deaminase (AID) that is encoded by the Aicda gene, and not in naive B cells that do not express AID. We first examined the efficiency of AID-Cre-mediated deletion of Ptpn6 f/f alleles by PCR analyses using genomic DNA from FACS-sorted activated (CD19 + CD38 − Fas + ) and non-activated (CD19 + CD38 + Fas − ) B cells from the Peyer’s patches (PP) of Ptpn6 f/f Aicda +/+ and Ptpn6 f/f Aicda Cre/+ mice ( Supplementary Fig. 1A ). Our results showed that the Ptpn6 f/f alleles were efficiently deleted in activated B cells from Ptpn6 f/f Aicda Cre/+ mice but remained intact in non-activated B cells from the same mice or in both activated and non-activated B cells from control Ptpn6 f/f Aicda +/+ mice ( Supplementary Fig. 1B ). This was further corroborated by flow cytometry analysis that revealed significant reduction in intracellular Shp1 protein level in activated B cells in Ptpn6 f/f Aicda Cre/+ mice compared with various controls ( Supplementary Fig. 1C ). Thus, Shp1 is specifically ablated in antigen-activated but not naive B cells in Ptpn6 f/f Aicda Cre/+ mice. We next examined B-cell development in unchallenged Ptpn6 f/f Aicda Cre/+ mice since it was reported previously that B-cell-specific ablation of Shp1 in Ptpn6 f/f CD19 Cre/+ mice led to skewed B-cell development in these animals [17] . Indeed, Ptpn6 f/f CD19 Cre/+ mice predominantly developed CD5 + B-1 cells in the spleen, lymph nodes and peritoneal cavity ( Fig. 1a ), exhibited defects in B-cell maturation in the periphery and bone marrow ( Fig. 1b ) and lacked follicular B cells in the spleen and lymph nodes ( Fig. 1c ). By contrast, Ptpn6 f/f Aicda Cre/+ mice had normal B lymphopoiesis in the bone marrow ( Fig. 1b ) and unperturbed B-cell subsets in the peritoneal cavity, spleen, and lymph nodes ( Fig. 1a–c ). Enumeration of B cells in Ptpn6 f/f Aicda Cre/+ mice also revealed that these mice had normal numbers of lymphocytes belonging to various B-cell subsets and were unlike Ptpn6 f/f CD19 Cre/+ mice that had decreased number of follicular B but exaggerated number of B-1 cells ( Fig. 1d ). In contrast to the disrupted splenic architecture seen in Ptpn6 f/f CD19 Cre/+ mice, histological examination also revealed normal compartmentalization of B and T cells in the splenic follicles of Ptpn6 f/f Aicda Cre/+ mice ( Fig. 1e ). Thus, taken together, Ptpn6 f/f Aicda Cre/+ mice exhibit normal bone marrow and peripheral B-cell development and present a better model to examine the role of Shp1 in B-cell terminal differentiation than Ptpn6 f/f CD19 Cre/+ mice that preferentially generate CD5 + B-1 cells and lack follicular B cells [17] . 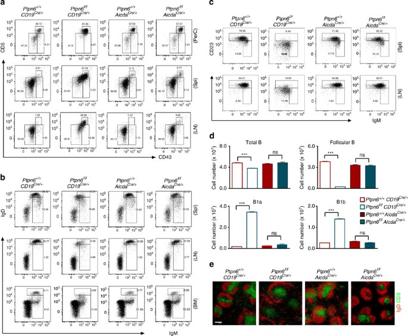Figure 1: Comparison of B-cell populations inPtpn6f/fCD19Cre/+andPtpn6f/fAicdaCre/+mice. Flow cytometric analyses of B-cell subsets in the peritoneal cavity (PerC), spleen (Spl), inguinal lymph nodes (LN) and bone marrow (BM) of mice of various genotypes. (a) Figure depicts CD19+B220+cells in various tissues stained for their expression of CD5 and CD43. B-1a (CD5+CD43+), B-1b (CD5−CD43+) and B-2 (CD5−CD43−) cells are indicated. Numbers indicate per cent of CD19+B220+cells. (b) Total Spl, LN and BM cells were stained for IgD and IgM expression and numbers adjacent to gated areas indicate per cent of CD19+cells. (c) CD19+cells in Spl and LN were gated for their expression of CD23 and IgM to delineate follicular (CD23+IgM+) and marginal zone (CD23−IgM+) B cells. Numbers indicate per cent of CD19+cells. (d) Enumeration of total B, follicular B, B-1a and B-1b cells in the spleens of mice of various genotypes, plotted as mean+s.e.m.;n=3, ***P<0.001 by two-tailed Student’st-test; ns=non-significant. (e) Spleen histology sections from mice of various genotypes. Frozen sections of spleen were stained with anti-IgD (red) and anti-CD3 (green) antibodies. One representative section out of three spleens per group examined is shown. White bar, 200 μm. Data shown ina–care representative of more than five independent analyses. Figure 1: Comparison of B-cell populations in Ptpn6 f/f CD19 Cre/+ and Ptpn6 f/f Aicda Cre/+ mice. Flow cytometric analyses of B-cell subsets in the peritoneal cavity (PerC), spleen (Spl), inguinal lymph nodes (LN) and bone marrow (BM) of mice of various genotypes. ( a ) Figure depicts CD19 + B220 + cells in various tissues stained for their expression of CD5 and CD43. B-1a (CD5 + CD43 + ), B-1b (CD5 − CD43 + ) and B-2 (CD5 − CD43 − ) cells are indicated. Numbers indicate per cent of CD19 + B220 + cells. ( b ) Total Spl, LN and BM cells were stained for IgD and IgM expression and numbers adjacent to gated areas indicate per cent of CD19 + cells. ( c ) CD19 + cells in Spl and LN were gated for their expression of CD23 and IgM to delineate follicular (CD23 + IgM + ) and marginal zone (CD23 − IgM + ) B cells. Numbers indicate per cent of CD19 + cells. ( d ) Enumeration of total B, follicular B, B-1a and B-1b cells in the spleens of mice of various genotypes, plotted as mean+s.e.m. ; n =3, *** P <0.001 by two-tailed Student’s t -test; ns=non-significant. ( e ) Spleen histology sections from mice of various genotypes. Frozen sections of spleen were stained with anti-IgD (red) and anti-CD3 (green) antibodies. One representative section out of three spleens per group examined is shown. White bar, 200 μm. Data shown in a – c are representative of more than five independent analyses. Full size image Lack of Shp1 signalling affects IgG1 antibody response To gain insight to the role of Shp1 in B-cell terminal differentiation, we immunized Ptpn6 +/+ Aicda Cre/+ and Ptpn6 f/f Aicda Cre/+ mice with alum-precipitated T-cell-dependent antigen, 4-hydroxy-3-nitrophenyl-acetyl (NP) coupled to chicken gamma-globulin (CGG) and examined their sera levels of NP-specific antibodies. The humoral immune response to NP-CGG is dominated by IgM and IgG1 antibodies [34] . Hence, we examined anti-NP IgM and IgG1 antibodies at 7, 14, 21 and 28 days post immunization ( Fig. 2a ). Interestingly, Ptpn6 f/f Aicda Cre/+ mice could produce equivalent titres of antigen-specific IgM but had defective production of IgG1 antibodies from day 14 onwards after primary immunization when compared with Ptpn6 +/+ Aicda Cre/+ mice. 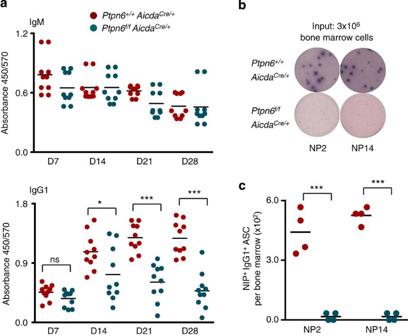Figure 2: Defective T-cell-dependent class-switched antibody response inPtpn6f/fAicdaCre/+mice. (a) Serum antigen-specific IgM and IgG1 antibody levels inPtpn6+/+AicdaCre/+(red circles) andPtpn6f/fAicdaCre/+(blue circles) mice examined at 7, 14, 21 and 28 days after primary immunization with NP38-CGG. Sera from mice were diluted 1,000 and 9,000 times, respectively, and measured via ELISA for the presence of anti-NP IgM and IgG1 antibodies. Data shown were representative of two independent experiments and each experimental group comprised 10 mice. (b) ELISPOT analyses and (c) enumeration of high-affinity (NP2) and total (NP14) anti-NP-specific IgG1 ASCs in the bone marrow ofPtpn6+/+AicdaCre/+andPtpn6f/fAicdaCre/+mice at 28 days post immunization. Data shown are representative of four independent experiments. Each circle represents one mouse analysed, *P<0.05 and ***P<0.001 by two-tailed Student’st-test; ns=non-significant. Figure 2: Defective T-cell-dependent class-switched antibody response in Ptpn6 f/f Aicda Cre/+ mice. ( a ) Serum antigen-specific IgM and IgG1 antibody levels in Ptpn6 +/+ Aicda Cre/+ (red circles) and Ptpn6 f/f Aicda Cre/+ (blue circles) mice examined at 7, 14, 21 and 28 days after primary immunization with NP 38 -CGG. Sera from mice were diluted 1,000 and 9,000 times, respectively, and measured via ELISA for the presence of anti-NP IgM and IgG1 antibodies. Data shown were representative of two independent experiments and each experimental group comprised 10 mice. ( b ) ELISPOT analyses and ( c ) enumeration of high-affinity (NP2) and total (NP14) anti-NP-specific IgG1 ASCs in the bone marrow of Ptpn6 +/+ Aicda Cre/+ and Ptpn6 f/f Aicda Cre/+ mice at 28 days post immunization. Data shown are representative of four independent experiments. Each circle represents one mouse analysed, * P <0.05 and *** P <0.001 by two-tailed Student’s t -test; ns=non-significant. Full size image Since immunized Ptpn6 f/f Aicda Cre/+ mice have impaired class-switched IgG1 antibody response, we further examined by ELISPOT whether ASCs were present in the bone marrow of these mice ( Fig. 2b ). At day 28 post immunization with NP 38 -CGG, we were able to detect a substantial number of high-affinity (NP2) and total (NP14) NP-specific IgG1 ASC in the bone marrow of control Ptpn6 +/+ Aicda Cre/+ mice. However, these ASCs were largely absent in the bone marrow of similarly immunized Ptpn6 f/f Aicda Cre/+ mice ( Fig. 2b,c ). We proceeded to re-challenge Ptpn6 f/f Aicda Cre/+ mice to assess their ability to mount a secondary response to the same antigen 30 days after primary challenge. As seen in Fig. 3a , control Ptpn6 +/+ Aicda Cre/+ mice mounted a robust recall response with much greater titres of antigen-specific IgG1 antibody at day 5 after secondary challenge but mutant mice still manifested defective response to the same antigen. ELISPOT analyses ( Fig. 3b ) and enumeration of ASCs ( Fig. 3c ) in the spleen and bone marrow of mice also indicated a deficit of ASC in Ptpn6 f/f Aicda Cre/+ compared with Ptpn6 +/+ Aicda Cre/+ mice. This observation was further corroborated by our histological examination, which revealed massive expansion of antigen-specific IgG1 ASC in the spleen of re-challenged Ptpn6 +/+ Aicda Cre/+ but not Ptpn6 f/f Aicda Cre/+ mice ( Fig. 3d ). 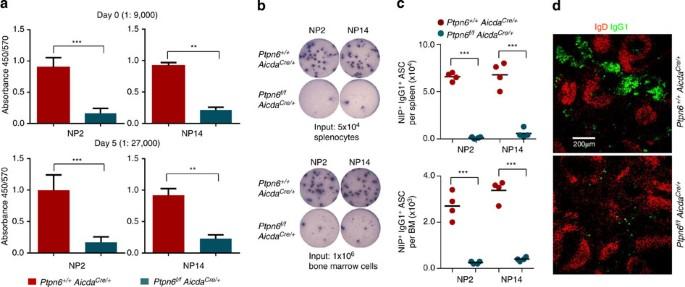Figure 3: Impaired antibody recalled response inPtpn6f/fAicdaCre/+mice. Mice previously immunized with NP38-CGG were re-challenged at day 30. (a) Antigen-specific IgG1 titres in the sera ofPtpn6+/+AicdaCre/+(red bars) andPtpn6f/fAicdaCre/+(blue bars) mice examined by ELISA at day 0 (1: 9,000 dilution) or day 5 (1: 27,000 dilution) of secondary immunization. (b) ELISPOT analyses of high affinity (NP2) and total (NP14) anti-NP ASC in the spleen (upper figure) and bone marrow (lower figure) of mice at day 5 after secondary challenge. (c) Enumeration of anti-NP ASC in the spleen and bone marrow of immunized mice. Each circle represents one single animal examined. Data shown are representative of three independent set of experiments and each experimental group comprised at least four mice. (d) Histological examination of IgG1 ASC in the spleen of mice at day 5 after re-challenge with NP38-CGG. Frozen sections of spleens were stained with anti-IgD (red) and anti-IgG1 (green) antibodies to reveal follicular B and PCs, respectively. Image shown is representative of four immunized spleens examined per mouse group. White bar, 200 μm, ***P<0.001 and **P<0.01 by two-tailed Student’st-test. Figure 3: Impaired antibody recalled response in Ptpn6 f/f Aicda Cre/+ mice. Mice previously immunized with NP 38 -CGG were re-challenged at day 30. ( a ) Antigen-specific IgG1 titres in the sera of Ptpn6 +/+ Aicda Cre/+ (red bars) and Ptpn6 f/f Aicda Cre/+ (blue bars) mice examined by ELISA at day 0 (1: 9,000 dilution) or day 5 (1: 27,000 dilution) of secondary immunization. ( b ) ELISPOT analyses of high affinity (NP2) and total (NP14) anti-NP ASC in the spleen (upper figure) and bone marrow (lower figure) of mice at day 5 after secondary challenge. ( c ) Enumeration of anti-NP ASC in the spleen and bone marrow of immunized mice. Each circle represents one single animal examined. Data shown are representative of three independent set of experiments and each experimental group comprised at least four mice. ( d ) Histological examination of IgG1 ASC in the spleen of mice at day 5 after re-challenge with NP 38 -CGG. Frozen sections of spleens were stained with anti-IgD (red) and anti-IgG1 (green) antibodies to reveal follicular B and PCs, respectively. Image shown is representative of four immunized spleens examined per mouse group. White bar, 200 μm, *** P <0.001 and ** P <0.01 by two-tailed Student’s t -test. Full size image Taken together, the data indicated that Ptpn6 f/f Aicda Cre/+ mice have defective primary and secondary T-cell-dependent antibody responses. This was quite unexpected as we would predict a heightened antibody response in immunized Ptpn6 f/f Aicda Cre/+ mice given that Shp1 is a negative regulator of B-cell-receptor signalling [5] . Instead, our current data suggest that Shp1 signalling during B-cell activation is required to generate effective humoral immunity. Shp1 signalling is critical for memory B-cell formation It is known that T-cell-dependent immune response elicits GC where antigen-activated B cells proliferate and give rise to memory B and long-lived PCs [35] . Our data above indicating defective T-cell-dependent antibody response in Ptpn6 f/f Aicda Cre/+ mice suggested that Shp1 might be important for GC formation and/or maintenance. Previous study using Ptpn6 f/f CD19 Cre/+ mice that also exhibited defective T-cell-dependent immune responses [17] did not address the role of Shp1 in GC B-cell differentiation. Moreover, the drastic reduction of follicular B-cell population in Ptpn6 f/f CD19 Cre/+ mice would render it difficult to study the role of Shp1 in GC formation. Recently, Shp1 was inducibly ablated in total B cells at the peak of an on-going T-cell-dependent immune response using tamoxifen-driven Cre and shown to affect GC maintenance [24] . However, a role for Shp1 signalling in GC B-cell formation has not been fully addressed. To resolve this issue, we analyse GC B cells in immunized Ptpn6 f/f Aicda Cre/+ mice. A first indication that Shp1 might not be required for GC B-cell formation arose from our observation of a sizeable fraction of CD19 + CD38 − Fas + B cells in the PP of Ptpn6 f/f Aicda Cre/+ mice that was indistinguishable from that found in Ptpn6 f/f Aicda +/+ mice ( Supplementary Fig. 1A ). However, PPs are sites of chronic antigenic stimulations and might not truly reflect bona fide GC reactions that arise in an acute antigen challenge. Hence, we examined GC formation in the spleens of NP 38 -CGG-immunized Ptpn6 f/f Aicda Cre/+ mice. At day 10 post immunization, both Ptpn6 +/+ Aicda Cre/+ and Ptpn6 f/f Aicda Cre/+ mice generated comparable fraction of CD19 + CD38 − Fas + GC B cells ( Fig. 4a,b ) and this was further corroborated by histological examination ( Fig. 4c ). Detailed analyses further revealed the presence of equivalent fraction of class-switched antigen-specific NIP + IgG1 + GC B cells in these mice ( Fig. 4d,e ). Hence, Shp1 signalling during B-cell activation is dispensable for the generation of GC B cells and its absence did not perturb or lead to exaggerated GC formation. 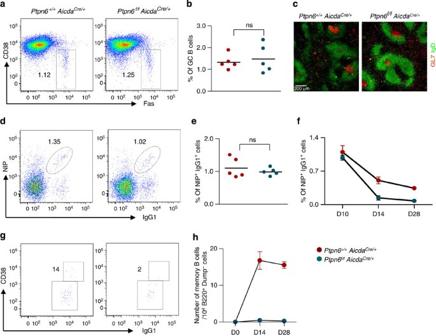Figure 4: Analyses of GC and memory B-cell formation inPtpn6f/fAicdaCre/+mice. Ptpn6+/+AicdaCre/+andPtpn6f/fAicdaCre/+mice were analysed 10 days onwards after challenge with NP38-CGG. (a) Flow cytometry analysis of CD19+cells in the spleens of immunized mice stained for the presence of Fas+CD38−GC B cells. Numbers indicate per cent of CD19+cells. (b) Graphical depiction of the frequencies of GC B cells in the spleens ofPtpn6+/+AicdaCre/+andPtpn6f/fAicdaCre/+mice. Each data point represents one mouse analysed and five mice per group were examined; ns=non-significant. (c) Histology staining of splenic GC with anti-IgD (green) and anti-GL7 (red) antibodies. White bar, 200 μm. (d) B220+Dump−cells in the spleens of immunized mice were analysed for the presence of antigen-specific NIP-binding IgG1 B cells. Numbers indicate per cent of IgG1 B cells in B220+Dump−gate that bind antigen. (e) Graphical representation of the frequencies of antigen-specific IgG1 cells in immunized spleens. (f) Graphical representation of the frequency of antigen-specific IgG1 cells at day 10, 14 and 28 post immunizations. Cells were gated as in (d). Group of five mice were used, and data are expressed as mean±s.e.m. (g) Flow cytometry analysis of NIP-binding IgG1 cells at day 14 of immunization to further delineate CD38−GC and CD38+memory B cells. Numbers indicate actual number of cells in the gated areas out of 104B220+Dump−spleen cells analysed. (h) Quantification of CD38+IgG1+NP-specific memory B cells (expressed as number of memory B cells per 104B220+Dump−cells) inPtpn6+/+AicdaCre/+andPtpn6f/fAicdaCre/+mice at 0, 14 and 28 days post immunizations. Group of five mice were used, and data are expressed as mean±s.e.m. Figure 4: Analyses of GC and memory B-cell formation in Ptpn6 f/f Aicda Cre/+ mice. Ptpn6 +/+ Aicda Cre/+ and Ptpn6 f/f Aicda Cre/+ mice were analysed 10 days onwards after challenge with NP 38 -CGG. ( a ) Flow cytometry analysis of CD19 + cells in the spleens of immunized mice stained for the presence of Fas + CD38 − GC B cells. Numbers indicate per cent of CD19 + cells. ( b ) Graphical depiction of the frequencies of GC B cells in the spleens of Ptpn6 +/+ Aicda Cre/+ and Ptpn6 f/f Aicda Cre/+ mice. Each data point represents one mouse analysed and five mice per group were examined; ns=non-significant. ( c ) Histology staining of splenic GC with anti-IgD (green) and anti-GL7 (red) antibodies. White bar, 200 μm. ( d ) B220 + Dump − cells in the spleens of immunized mice were analysed for the presence of antigen-specific NIP-binding IgG1 B cells. Numbers indicate per cent of IgG1 B cells in B220 + Dump − gate that bind antigen. ( e ) Graphical representation of the frequencies of antigen-specific IgG1 cells in immunized spleens. ( f ) Graphical representation of the frequency of antigen-specific IgG1 cells at day 10, 14 and 28 post immunizations. Cells were gated as in ( d ). Group of five mice were used, and data are expressed as mean±s.e.m. ( g ) Flow cytometry analysis of NIP-binding IgG1 cells at day 14 of immunization to further delineate CD38 − GC and CD38 + memory B cells. Numbers indicate actual number of cells in the gated areas out of 10 4 B220 + Dump − spleen cells analysed. ( h ) Quantification of CD38 + IgG1 + NP-specific memory B cells (expressed as number of memory B cells per 10 4 B220 + Dump − cells) in Ptpn6 +/+ Aicda Cre/+ and Ptpn6 f/f Aicda Cre/+ mice at 0, 14 and 28 days post immunizations. Group of five mice were used, and data are expressed as mean±s.e.m. Full size image To reconcile previous work demonstrating that Shp1 played a role in GC maintenance [24] and our data above indicating that Shp1 in activated B cells was not required to generate GC B cells, we tracked the frequencies of NIP + IgG1 + GC B cells in Ptpn6 f/f Aicda Cre/+ mice at various time-points post immunization. At day 10 of antigenic challenge when GC began to form, Ptpn6 +/+ Aicda Cre/+ and Ptpn6 f/f Aicda Cre/+ mice generated equivalent frequencies of antigen-specific GC B cells. However, the frequencies of GC B cells decreased much more rapidly with time in immunized Ptpn6 f/f Aicda Cre/+ compared with Ptpn6 +/+ Aicda Cre/+ mice ( Fig. 4f ), suggesting that GC maintenance is compromised in these mice and this is consistent with previous finding. We also studied the formation of B-cell memory by examining the presence of CD38 + NIP + IgG1 + memory B cells in immunized Ptpn6 f/f Aicda Cre/+ mice at various time-points post immunization. A significant number of memory B cells can be detected at day 14 ( Fig. 4g ) and they persist to day 28 post antigenic challenge in Ptpn6 +/+ Aicda Cre/+ mice ( Fig. 4h ). However, memory B cells were barely detectable at both time-points in immunized Ptpn6 f/f Aicda Cre/+ mice, suggesting that these cells were not formed. Taken together, our data indicated that Shp1 signalling during B-cell activation is important to sustain GC reaction and to generate memory B cells and their impairments could account for the compromised T-cell-dependent recall response seen in these mice. Shp1-deficient PCs are not found in the bone marrow Since NIP + IgG1 + GC B cells were present at day 10 ( Fig. 4d ) and yet no long-lived PC was detected in the bone marrow at day 28 ( Fig. 2b ) of antigen-challenged Ptpn6 f/f Aicda Cre/+ mice, we proceeded to determine whether antigen-activated B cells lacking Shp1 could generate PCs given that they could not generate memory B cells. PCs are thought to arise in the spleen and other peripheral lymphoid tissues and migrate to the bone marrow to form the long-lived pool [21] , [22] . Thus, we examined NP-specific IgG1 ASC in the spleen of antigen-challenged Ptpn6 f/f Aicda Cre/+ mice at an early time-point in the immunization regime. Interestingly, at day 14 post immunization, we were able to detect by ELISPOT equivalent numbers of NP-specific IgG1 ASC in the spleen of Ptpn6 f/f Aicda Cre/+ mice compared with control Ptpn6 +/+ Aicda Cre/+ mice ( Fig. 5a ). However, the number of ASC was drastically reduced in the bone marrow of Ptpn6 f/f Aicda Cre/+ mice ( Fig. 5b ). Histological examination of tissue section at day 14 post immunization confirmed the presence of IgG1 ASC in the spleen of immunized Ptpn6 f/f Aicda Cre/+ mice but these cells were scattered spatially ( Fig. 5c ) and unlike the ASCs found in the spleen of Ptpn6 +/+ Aicda Cre/+ mice that were found in clusters in the extrafollicular space. These data together suggested that antigen-activated B cells lacking Shp1 could differentiate into PCs at the site of activation, but for yet-to-be determined reasons, could not form the long-lived PC pool in the bone marrow. 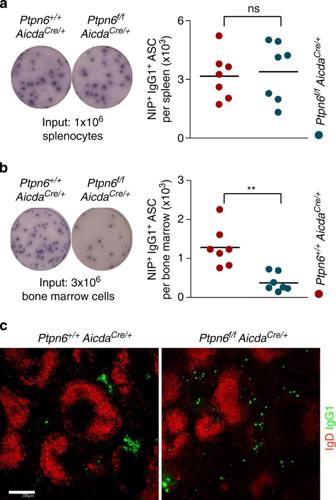Figure 5: Reduced ASC numbers in the bone marrow but not spleen of immunizedPtpn6f/fAicdaCre/+mice. ELISPOT analyses and quantification of anti-NP IgG1 ASC in the spleen (a) and bone marrow (b) ofPtpn6+/+AicdaCre/+(red circles) andPtpn6f/fAicdaCre/+(blue circles) mice at day 14 after primary immunization with NP38-CGG. Each circle represents one mouse examined; **P<0.01 by two-tailed Student’st-test; ns=non-significant. (c) Confocal immunoflorescence microscopy analyses of frozen spleen sections from NP38-CGG-immunizedPtpn6+/+AicdaCre/+andPtpn6f/fAicdaCre/+mice. Spleen sections were stained with anti-IgD (red) and anti-IgG1 (green) antibodies. Image shown is representative of three spleens per group examined. White bar, 200 μm. Figure 5: Reduced ASC numbers in the bone marrow but not spleen of immunized Ptpn6 f/f Aicda Cre/+ mice. ELISPOT analyses and quantification of anti-NP IgG1 ASC in the spleen ( a ) and bone marrow ( b ) of Ptpn6 +/+ Aicda Cre/+ (red circles) and Ptpn6 f/f Aicda Cre/+ (blue circles) mice at day 14 after primary immunization with NP 38 -CGG. Each circle represents one mouse examined; ** P <0.01 by two-tailed Student’s t -test; ns=non-significant. ( c ) Confocal immunoflorescence microscopy analyses of frozen spleen sections from NP 38 -CGG-immunized Ptpn6 +/+ Aicda Cre/+ and Ptpn6 f/f Aicda Cre/+ mice. Spleen sections were stained with anti-IgD (red) and anti-IgG1 (green) antibodies. Image shown is representative of three spleens per group examined. White bar, 200 μm. Full size image Enhanced α4β1 activation in PCs lacking Shp1 The presence of ASC in the spleen at day 14 and their absence in the bone marrow at days 14 and 28 of immunized Ptpn6 f/f Aicda Cre/+ mice prompted us to query whether mutant ASC have homing defects. Our histological analysis showing a lack of clustering of PCs in Ptpn6 f/f Aicda Cre/+ mice ( Fig. 5c ) yielded the first hint that these cells might have altered adhesion and chemotactic properties. It is known that the homing of PC to bone marrow is highly dependent on the function of chemokine receptors and integrins [21] , [22] . Previous reports have shown that chemokine receptors and integrins are abundantly expressed on ASC [27] , [30] , [36] and the loss of chemokine receptor or integrin is known to lead to defective egress of ASC from lymphoid organs [25] , [36] , [37] . Hence, we examine the expression and function of chemokine receptor and integrins on ASC. We immunized Ptpn6 +/+ Aicda Cre/+ and Ptpn6 f/f Aicda Cre/+ mice to generate PC in vivo . The gating strategy for plasma (B220 low CD138 + ) and non-plasma (B220 + CD138 − ) cells in immunized mice was depicted in Fig. 6a . We first assessed the expression level of chemokine receptor CXCR4, which is known to regulate PC homing [36] and found them to be comparable between Ptpn6 +/+ Aicda Cre/+ and Ptpn6 f/f Aicda Cre/+ mice ( Supplementary Fig. 2A ). In addition, Shp1-deficient cells displayed similar responsiveness to CXCR4 ligand, SDF-1α ( Supplementary Fig. 2B ). These data indicated that CXCR4 signalling remains intact in Shp1-deficient ASC. 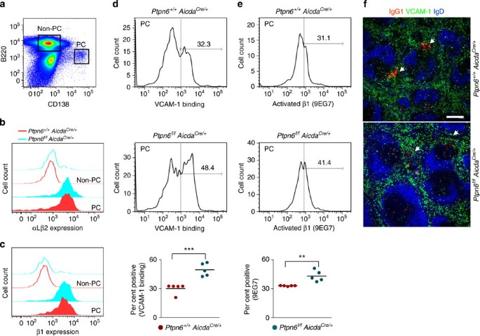Figure 6: Shp1-deficient PCs manifest enhanced α4β1 integrin-binding affinity. PCs from mice challenged with NP38-CGG were analysed at day 10 post immunization for the expression and activation of adhesion molecules. (a) Flow cytometry figure depicts gating strategy for splenic PC (B220lowCD138+) and non-PCs (non-PC, B220+CD138−) from immunized mice. Flow cytometry analyses of (b) αLβ2 and (c) β1 integrin expression on PC (shaded histogram) and non-PC (unshaded histogram) from immunizedPtpn6+/+AicdaCre/+(red histogram) andPtpn6f/fAicdaCre/+(blue histogram) mice. Histograms were overlaid for direct comparison. (d) Binding of soluble VCAM-1-Fc (20 μg ml−1) by PC from immunizedPtpn6+/+AicdaCre/+(upper panel) orPtpn6f/fAicdaCre/+(middle panel) mice and quantification of the percentage of VCAM-1-binding PCs (lower panel) in these mice. (e) Flow cytometry staining of PC from immunizedPtpn6+/+AicdaCre/+(upper panel) andPtpn6f/fAicdaCre/+(middle panel) mice with the 9EG7 antibody and quantification (lower panel) of the percentage of 9EG7-positive PC in these mice. Each circle represented one mouse analysed and **P<0.01 by two-tailed Student’st-test. (f) Frozen spleen sections from NP38-CGG-immunizedPtpn6+/+AicdaCre/+andPtpn6f/fAicdaCre/+mice were stained with anti-IgD (blue), anti-IgG1 (red) and anti-VCAM-1 (green) antibodies and analysed by confocal microscopy. Image shown is representative of three spleen sections per group examined. White bar, 200 μm. Figure 6: Shp1-deficient PCs manifest enhanced α4β1 integrin-binding affinity. PCs from mice challenged with NP 38 -CGG were analysed at day 10 post immunization for the expression and activation of adhesion molecules. ( a ) Flow cytometry figure depicts gating strategy for splenic PC (B220 low CD138 + ) and non-PCs (non-PC, B220 + CD138 − ) from immunized mice. Flow cytometry analyses of ( b ) αLβ2 and ( c ) β1 integrin expression on PC (shaded histogram) and non-PC (unshaded histogram) from immunized Ptpn6 +/+ Aicda Cre/+ (red histogram) and Ptpn6 f/f Aicda Cre/+ (blue histogram) mice. Histograms were overlaid for direct comparison. ( d ) Binding of soluble VCAM-1-Fc (20 μg ml −1 ) by PC from immunized Ptpn6 +/+ Aicda Cre/+ (upper panel) or Ptpn6 f/f Aicda Cre/+ (middle panel) mice and quantification of the percentage of VCAM-1-binding PCs (lower panel) in these mice. ( e ) Flow cytometry staining of PC from immunized Ptpn6 +/+ Aicda Cre/+ (upper panel) and Ptpn6 f/f Aicda Cre/+ (middle panel) mice with the 9EG7 antibody and quantification (lower panel) of the percentage of 9EG7-positive PC in these mice. Each circle represented one mouse analysed and ** P <0.01 by two-tailed Student’s t -test. ( f ) Frozen spleen sections from NP 38 -CGG-immunized Ptpn6 +/+ Aicda Cre/+ and Ptpn6 f/f Aicda Cre/+ mice were stained with anti-IgD (blue), anti-IgG1 (red) and anti-VCAM-1 (green) antibodies and analysed by confocal microscopy. Image shown is representative of three spleen sections per group examined. White bar, 200 μm. Full size image We next studied the expression of αLβ2 ( Fig. 6b ) and α4β1 ( Fig. 6c ) integrins and found PCs from Ptpn6 f/f Aicda Cre/+ mice to be able to upregulate the expression of these molecules to the same extent as PCs from Ptpn6 +/+ Aicda Cre/+ mice. Thus, integrin expression levels could not account for the drastic reduction of ASCs in the bone marrow of Ptpn6 f/f Aicda Cre/+ mice. Other than regulation at the expression levels, integrins are known to change their affinity states, through inside-out and outside-in signalling pathways, to bind their ligands [38] , [39] . They undergo rapid activation and deactivation upon cell stimulation. The integrin ligands ICAM-1 and VCAM-1 are abundantly expressed in splenic red pulps, which are exit sites for PCs [40] . Shp1 has been implicated in the negative regulation of integrin activation in macrophages and neutrophils [10] , [11] . This led us to postulate that Shp1-deficient PCs might also have altered integrin activation. We first determined whether Shp1-deficient PCs have altered αLβ2 activity by examining its binding of the ligand ICAM-1 ( Supplementary Fig. 3A ). To our surprise, mutant PCs exhibited equivalent binding of ICAM-1 as wild-type PC, suggesting that Shp1-deficient PCs have normal αLβ2 activation. We next examined the affinity status of α4β1 integrin, as high-affinity α4β1 binds to VCAM-1 (ref. 41 ). Interestingly, we noted that Shp1-deficient PCs had enhanced α4β1 binding to soluble VCAM-1 when compared with control PC ( Fig. 6d ). By contrast, Shp1-deficient non-PC B cells did not display any altered α4β1 binding activity towards VCAM-1 ( Supplementary Fig. 3B ), suggesting that the phenomenon occurred only in PCs. To confirm our observation, we employed an activation-specific antibody 9EG7 to examine the activation status of α4β1 in PCs from control and Ptpn6 f/f Aicda Cre/+ mice ( Fig. 6e ). Again, Shp1-deficient PCs displayed greater staining with the 9EG7 antibody, which recognized an activated epitope of α4β1. Histological staining indicated that VCAM-1 was widely expressed in the extrafollicular space where PC clustered in wild-type animals but scattered in the mutant mice, presumably due to enhanced adhesive property of the mutant cells, which prevented them from migrating to and congregating at exit points in the spleen ( Fig. 6f ). Taken together, our data indicated that Shp1-deficiency leads specifically to higher binding affinity of α4β1 integrin and suggested that Shp1 could be involved in regulating the activation of α4β1 integrin on PCs. Shp1-deficient PC have reduced migratory properties Owing to the limited number of PCs that we could recover from mice ex vivo , we used in vitro LPS-differentiated PCs for in-depth characterization of the role of Shp1 in PC physiology. First of all, we examined the activation status of Shp1 in PC vis-à-vis non-PC to determine whether Shp1 plays a role in this late stage of B-cell differentiation. To this end, we FACS-sorted wild-type PC (B220 low CD138 + ) and non-PC (B220 + CD138 − ) and examined the phosphorylation status of Shp1 in these cells using a phospho-Shp1 specific antibody. We found Shp1 phosphorylation and hence activation to be significantly enhanced in PC compared with non-PC cells ( Fig. 7a , Supplementary Fig. 6 ). This finding suggested that activated Shp1 likely plays an important role in PC biology. 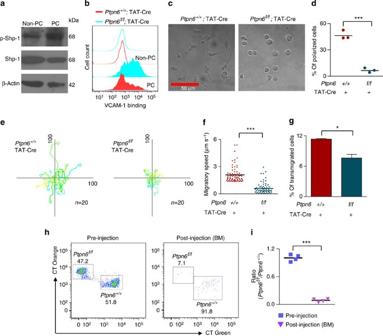Figure 7: Shp1-deficient PCs exhibit attenuated motility and impaired homing to bone marrow. (a) Shp1 is highly phosphorylated in PC. Purified wild-type B cells were stimulated with LPS (20 μg ml−1) for 3 days and PC (B220lowCD138+) and non-PC (B220+CD138−) fractions were FACS-sorted and analysed via western blotting with antibodies that bind phospho-Shp1 (Y564). The total Shp1 and β-actin blots act as loading controls. (b) Flow cytometry analyses of soluble VCAM-1-Fc binding byin vitroTat-Cre-transduced, LPS-differentiated PC fromPtpn6+/+(red shaded histogram) andPtpn6f/f(blue shaded histogram) mice. VCAM-1 binding by non-PC fromPtpn6+/+(red unshaded histogram) andPtpn6f/f(blue unshaded histogram) mice were also examined and overlaid for comparison. (c) Representative microscopic image showing the morphology of Tat-Cre-transduced, LPS-stimulatedPtpn6+/+andPtpn6f/fcells incubated for 15 min in the presence of 20 μg ml−1immobilized VCAM-1-Fc. Red bar, 50 μm. (d) Quantification of the percentage of polarized cells in (c), each dot represents data from an independent set of experiment and ***P<0.001 by two-tailed Student’st-test. (e) Superimposed image of the migratory paths of Tat-Cre-transduced, LPS-stimulatedPtpn6+/+andPtpn6f/fB cells. Image is collated from 20 randomly selected cells monitored over 30 min tracks with starting co-ordinates placed at the origin and movement documented in thexyplane. Each line represents the migratory path of one single cell. (f) Quantification of the migratory speed of Tat-Cre-transduced, LPS-stimulatedPtpn6+/+andPtpn6f/fB cells in the presence of 20 μg ml−1immobilized VCAM-1-Fc. Each dot represents one cell monitored, ***P<0.001 by two-tailed Student’st-test. (g) Transmigration of FACS-sortedPtpn6+/+andPtpn6f/fPCs through a VCAM-1-Fc (40 μg ml−1) coated trans-well with lower chamber containing 2 μg ml−1SDF-1α,n=3 and *P<0.05 by two-tailed Student’st-test. (h,i) B cells that were Tat-Cre-transduced and LPS-stimulated were labelled with CT-Green (Ptpn6+/+) and CT Orange (Ptpn6f/f) and reconstituted into wild-type mice. FACS analyses and statistic of cell mixture pre-injection (h, left) and 16 h post-injection (bone marrow,h, right). Ratio ofPtpn6f/ftoPtpn6+/+PCs before (≈1) and post (≈0.088) reconstitution were shown. Each data point refers to one set of experiment. Figure 7: Shp1-deficient PCs exhibit attenuated motility and impaired homing to bone marrow. ( a ) Shp1 is highly phosphorylated in PC. Purified wild-type B cells were stimulated with LPS (20 μg ml −1 ) for 3 days and PC (B220 low CD138 + ) and non-PC (B220 + CD138 − ) fractions were FACS-sorted and analysed via western blotting with antibodies that bind phospho-Shp1 (Y564). The total Shp1 and β-actin blots act as loading controls. ( b ) Flow cytometry analyses of soluble VCAM-1-Fc binding by in vitro Tat-Cre-transduced, LPS-differentiated PC from Ptpn6 +/+ (red shaded histogram) and Ptpn6 f/f (blue shaded histogram) mice. VCAM-1 binding by non-PC from Ptpn6 +/+ (red unshaded histogram) and Ptpn6 f/f (blue unshaded histogram) mice were also examined and overlaid for comparison. ( c ) Representative microscopic image showing the morphology of Tat-Cre-transduced, LPS-stimulated Ptpn6 +/+ and Ptpn6 f/f cells incubated for 15 min in the presence of 20 μg ml −1 immobilized VCAM-1-Fc. Red bar, 50 μm. ( d ) Quantification of the percentage of polarized cells in ( c ), each dot represents data from an independent set of experiment and *** P <0.001 by two-tailed Student’s t -test. ( e ) Superimposed image of the migratory paths of Tat-Cre-transduced, LPS-stimulated Ptpn6 +/+ and Ptpn6 f/f B cells. Image is collated from 20 randomly selected cells monitored over 30 min tracks with starting co-ordinates placed at the origin and movement documented in the xy plane. Each line represents the migratory path of one single cell. ( f ) Quantification of the migratory speed of Tat-Cre-transduced, LPS-stimulated Ptpn6 +/+ and Ptpn6 f/f B cells in the presence of 20 μg ml −1 immobilized VCAM-1-Fc. Each dot represents one cell monitored, *** P <0.001 by two-tailed Student’s t -test. ( g ) Transmigration of FACS-sorted Ptpn6 +/+ and Ptpn6 f/f PCs through a VCAM-1-Fc (40 μg ml −1 ) coated trans-well with lower chamber containing 2 μg ml −1 SDF-1α, n =3 and * P <0.05 by two-tailed Student’s t -test. ( h , i ) B cells that were Tat-Cre-transduced and LPS-stimulated were labelled with CT-Green ( Ptpn6 +/+ ) and CT Orange ( Ptpn6 f/f ) and reconstituted into wild-type mice. FACS analyses and statistic of cell mixture pre-injection ( h , left) and 16 h post-injection (bone marrow, h , right). Ratio of Ptpn6 f/f to Ptpn6 +/+ PCs before (≈1) and post (≈0.088) reconstitution were shown. Each data point refers to one set of experiment. Full size image Since antigen-specific PC could be generated in immunized Ptpn6 f/f Aicda Cre/+ mice, we investigated whether Shp1-deficient PCs could also be generated in vitro . To address this question, we transduced Tat-Cre into Ptpn6 +/+ and Ptpn6 f/f B cells and stimulated them with LPS for 3 days. Flow cytometry analysis indicated that we were able to generate equivalent fractions of B220 low CD138 + PC from both cultures ( Supplementary Fig. 4A ) and further analyses by qRT–PCR ( Supplementary Fig. 4B ) and western blotting ( Supplementary Fig. 4C ) indicated that Shp1 was efficiently ablated in PC obtained from Tat-Cre-transduced and LPS-stimulated Ptpn6 f/f but not Ptpn6 +/+ cells. Taken together, the data indicated that Shp1-deficient plasmablasts can be generated in vitro , further confirming that Shp1 is not required for PC generation per se . We next examined whether the in vitro generated Shp1-deficient PC would also exhibit enhanced α4β1 binding affinity for VCAM-1. As shown in Fig. 7b and compared with Shp1-deficient non-PC or Shp1-sufficient cells, Shp1-deficient PC displayed enhanced binding of soluble VCAM-1. These data indicated that the in vitro generated Shp1-deficient PC recapitulated the behaviour of in vivo Shp1-deficient PC. Previous studies have shown that intact α4β1 integrin signalling is required for the migration of lymphocytes [42] , [43] , and failure of deactivation of this integrin leads to impaired cell migration [44] . Given that Shp1-deficient PC displayed enhanced activation of α4β1 integrin, we were keen to elucidate the effect of α4β1 hyperactivation on the migration of Shp1-deficient cells. We used videomicroscopy to map the migration of Shp1-sufficient and -deficient cells on VCAM-1-coated surfaces. First of all, we noticed that as cells moved on VCAM-1-coated surfaces, LPS-differentiated Shp1-sufficient cells displayed highly elongated and polarized morphology ( Fig. 7c ), which is known to be a prerequisite for cell migration [45] , [46] , [47] . Detailed analysis revealed that a significant number of Shp1-sufficient cells displayed elongated morphology, but Shp1-deficient cells were mostly rounded ( Fig. 7c,d ). Cell tracking analysis further revealed that Shp1-deficient cells displayed limited migration ( Fig. 7e ) and had reduced migratory speed ( Fig. 7f ). Shp1-deficient PCs were also impaired in their capacity to transmigrate through VCAM-1-coated trans-wells ( Fig. 7g ). Taken together, the in vitro data suggested that Shp1 signalling might be important for PC migration. Shp1-deficient PC have defects in bone marrow homing To further investigate the effect of enhanced adhesion and attenuated migration of Shp1-deficient PC on their homing to bone marrow in vivo , we introduced intravenously, equal number of differentially fluorescence-labelled LPS-activated Shp1-sufficient and -deficient B cells into wild-type recipient mice ( Fig. 7h ). Flow cytometry analysis of reconstituted mice revealed the presence of Shp1-sufficient PC in the bone marrow but Shp1-deficient PCs were conspicuously absent ( Fig. 7h,i ). Thus, the data suggested that Shp1 signalling is important for PC homing to the bone marrow. We next investigated whether the enhanced adhesive property due to aberrant α4β1 integrin activation was the underlying cause for the defective bone marrow homing of Shp1-deficient PC. To this end, we blocked α4β1 interaction with VCAM-1 in immunized Ptpn6 f/f Aicda Cre/+ mice. Ptpn6 +/+ Aicda Cre/+ and Ptpn6 f/f Aicda Cre/+ mice were immunized with alum-precipitated NP 38 -CGG and 10 days later, given isotype-matched control antibody, or further in the case of immunized Ptpn6 f/f Aicda Cre/+ mice, anti-VCAM-1 antibody. At day 14 post immunization (4 days post anti-VCAM-1 or control antibody treatment), we were able to detect by ELISPOT equivalent numbers of NP-specific IgG1 ASC in the spleens of Ptpn6 f/f Aicda Cre/+ and Ptpn6 +/+ Aicda Cre/+ mice, with or without anti-VCAM-1 antibody treatment ( Fig. 8a,b ). In agreement with previous data, the number of ASC was drastically reduced in the bone marrow of immunized Ptpn6 f/f Aicda Cre/+ mice given control antibody compared with similarly treated Ptpn6 +/+ Aicda Cre/+ mice ( Fig. 8c ). Interestingly, however, the number of ASC was significantly greater in the bone marrow of Ptpn6 f/f Aicda Cre/+ mice after anti-VCAM-1 antibody treatment ( Fig. 8c,d ). Hence, the result suggested that blocking α4β1–VCAM-1 interaction in immunized Ptpn6 f/f Aicda Cre/+ mice led to greater number of Shp1-deficient PC homing to the bone marrow. 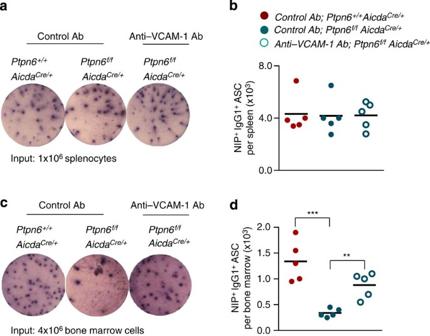Figure 8:In vivoblockage of α4β1–VCAM-1 interaction rectified bone marrow homing defect of Shp1-deficient PC. Mice immunized with NP38-CGG were i.v. injected with 100 μg isotype-matched control or anti-VCAM-1 antibody at day 10 post immunization. ELISPOT analyses and quantification of anti-NP IgG1 ASC in the spleen (a,b) and bone marrow (c,d) ofPtpn6+/+AicdaCre/+(red) andPtpn6f/fAicdaCre/+(blue) mice at day 14 post immunization. Each circle represents one mouse examined; ***P<0.001 and **P<0.01 by two-tailed Student’st-test. Figure 8: In vivo blockage of α4β1–VCAM-1 interaction rectified bone marrow homing defect of Shp1-deficient PC. Mice immunized with NP 38 -CGG were i.v. injected with 100 μg isotype-matched control or anti-VCAM-1 antibody at day 10 post immunization. ELISPOT analyses and quantification of anti-NP IgG1 ASC in the spleen ( a , b ) and bone marrow ( c , d ) of Ptpn6 +/+ Aicda Cre/+ (red) and Ptpn6 f/f Aicda Cre/+ (blue) mice at day 14 post immunization. Each circle represents one mouse examined; *** P <0.001 and ** P <0.01 by two-tailed Student’s t -test. Full size image Enhanced Src- and PI3-kinase signalling in Shp1-deficient PCs Shp1 has been shown to directly associate with the cytoplasmic tails of integrins [32] , [33] , which signal through various intracellular protein kinases, including Src family kinase and phosphoinositide-3 kinase (PI3-kinase) [48] . To determine whether the activation of these kinases was affected by Shp1 deficiency in PCs, we sorted PCs (B220 low CD138 + ) from Tat-Cre-transduced, LPS-differentiated Ptpn6 +/+ and Ptpn6 f/f cell cultures and found both Src family kinase and PI3-kinase to be hyperphosphorylated in Shp1-deficient cells ( Fig. 9a , Supplementary Fig. 6 ). The hyperactivation of PI3-kinase in Shp1-deficient PC was further confirmed by phospho-flow experiment showing enhanced phosphorylation of its downstream substrate, AKT ( Fig. 9b ). By contrast, the activation of Syk and ERK kinases were not altered in Shp1-deficient PC ( Supplementary Fig. 5 ), thus indicating that Shp1 deficiency selectively impaired distinct signalling pathways. 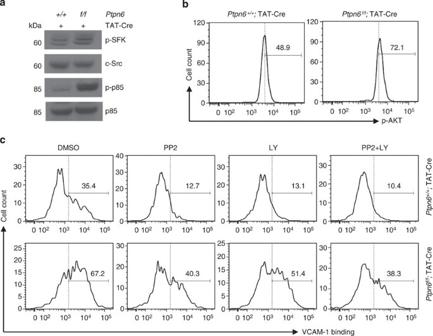Figure 9: PCs lacking Shp1 have enhanced Src family kinase and PI3-kinase signalling. Purified splenic B cells fromPtpn6+/+andPtpn6f/fmice were transduced with Tat-Cre and stimulated with LPS for 3 days to differentiate PCs. (a) Immunoblot analyses of Src family kinase (SFK) and PI3-kinase activation in FACS-sorted PC using anti-phospho-SFK and anti-phospho-p85α-specific antibodies (diluted 1:1,000 in 5% BSA in TBST). The anti-c-Src and anti-p85 blots served as loading controls. (b) Flow cytometry analysis of phospho-AKT content in gated B220lowCD138+PC fractions from Tat-Cre-transduced LPS-stimulatedPtpn6+/+(left panel) andPtpn6f/f(right panel) B cells. (c) Flow cytometry analyses of soluble VCAM-1-Fc binding by Tat-Cre-transduced, LPS-differentiated PC fromPtpn6+/+(upper panel) orPtpn6f/fcells (lower panel) in the presence of DMSO (solvent), PP2 (inhibitor of SFK; 10 μM) or LY294002 (inhibitor of PI3-kinase; 10 μM) or both together. Numbers indicate percentage of PCs that bind VCAM-1. Figure 9: PCs lacking Shp1 have enhanced Src family kinase and PI3-kinase signalling. Purified splenic B cells from Ptpn6 +/+ and Ptpn6 f/f mice were transduced with Tat-Cre and stimulated with LPS for 3 days to differentiate PCs. ( a ) Immunoblot analyses of Src family kinase (SFK) and PI3-kinase activation in FACS-sorted PC using anti-phospho-SFK and anti-phospho-p85α-specific antibodies (diluted 1:1,000 in 5% BSA in TBST). The anti-c-Src and anti-p85 blots served as loading controls. ( b ) Flow cytometry analysis of phospho-AKT content in gated B220 low CD138 + PC fractions from Tat-Cre-transduced LPS-stimulated Ptpn6 +/+ (left panel) and Ptpn6 f/f (right panel) B cells. ( c ) Flow cytometry analyses of soluble VCAM-1-Fc binding by Tat-Cre-transduced, LPS-differentiated PC from Ptpn6 +/+ (upper panel) or Ptpn6 f/f cells (lower panel) in the presence of DMSO (solvent), PP2 (inhibitor of SFK; 10 μM) or LY294002 (inhibitor of PI3-kinase; 10 μM) or both together. Numbers indicate percentage of PCs that bind VCAM-1. Full size image To determine whether the increased binding of VCAM-1 by α4β1 integrin in Shp1-deficient PC was a result of enhanced activation of Src and/or PI3-kinase, we treated Tat-Cre-transduced, LPS-differentiated Ptpn6 +/+ and Ptpn6 f/f B cells with chemical inhibitors to these kinases ( Fig. 9c ) and subsequently assessed their binding of soluble VCAM-1. Consistent with previous ex vivo observation, in vitro generated Shp1-deficient PCs exhibited enhanced binding of VCAM-1 compared with control cells and this binding of VCAM-1 by Ptpn6 f/f cells could be downmodulated to the levels seen in the wild-type counterparts by treatment with either Src kinase inhibitor PP2 or PI3-kinase inhibitor LY294002 or both together. These data together imply that the absence of Shp1 in PCs resulted in the hyperactivation of Src and PI3-kinase that subsequently led to increased α4β1 binding affinity for VCAM-1, and the impairment of PC migration to the bone marrow. Here, we generated Ptpn6 f/f Aicda Cre/+ mice and demonstrated that they have normal B-cell development in their bone marrow and peripheral lymphoid organs and the mice display normal splenic architecture before challenge with antigen. This is unlike the skewed generation of CD5 + B-1 cells and disrupted splenic follicles seen in motheaten [49] or Ptpn6 f/f CD19 Cre/+ (ref. 17 ) mice that have total or B-cell-specific Shp1 ablation, respectively. Thus, Ptpn6 f/f Aicda Cre/+ mice present a better mouse model to study the role of Shp1 in naive follicular B-cell terminal differentiation. When immunized Ptpn6 f/f Aicda Cre/+ mice were examined for the presence of antigen-specific antibodies in their sera, they were found to be defective. This was surprising as one would predict a heightened response given that Shp1 acts to downregulate activation and in its absence, there should be increased or sustained PC activation leading to greater antibody production and in line with the autoimmune phenotype seen in motheaten mice. When immunized Ptpn6 f/f Aicda Cre/+ mice were re-challenged with the same antigen, the recall antibody response was also severely compromised. Our detailed analyses revealed that while Ptpn6 f/f Aicda Cre/+ mice could generate GC B cells, these cells could not persist and this was consistent with previous finding [24] . Interestingly, memory B cells were not formed. Thus the absence of Shp1 impaired the development of B-cell memory. The defective antibody response also prompted us to examine the long-lived bone marrow PC pool in Ptpn6 f/f Aicda Cre/+ mice. Interestingly, ASC could be formed at early time-points in the spleens of immunized Ptpn6 f/f Aicda Cre/+ mice, indicating that unlike memory B cells, Shp1 is not required for the generation of PCs per se . This observation was further confirmed in vitro in LPS-stimulated cultures. However, no long-lived PCs were found in the bone marrow of immunized Ptpn6 f/f Aicda Cre/+ mice. The combined absence of memory B cells and long-lived PC in Ptpn6 f/f Aicda Cre/+ mice could explain why these mice have severely compromised recall humoral response. Since Shp1-deficient PC could be found in the spleens at early time-points during antigenic challenge but are absent in the long-lived pool in the bone marrow of immunized Ptpn6 f/f Aicda Cre/+ mice, it is likely that Shp1-deficient PC have a homing defect. Adhesion molecules are important for the proper localization of PC. For example, α4β7 integrin is critical for IgA-secreting cells to home to the gut [50] , [51] . Spleen-derived IgG ASC are known to highly express α4β1 and αLβ2 integrins, both of which are important for bone marrow homing [21] , [22] . Loss of integrin subunit α4 or β2 has been shown to impair cell homing to the bone marrow [25] , [52] . In addition, VCAM-1, which is the ligand for α4β1 integrin, is also needed for cell homing to bone marrow [31] , [53] . Aside from expression changes, the activation and deactivation of adhesion molecules also affect lymphocyte homing and could affect humoral response [44] , [54] . We found Shp1-deficient PC to be able to upregulate and express normal levels of α4β1 and αLβ2 integrins. Interestingly, Shp1-deficient PC have heightened activation of α4β1 but not αLβ2 integrins as evidenced by their binding to VCAM-1 and ICAM-1, respectively. Thus, we show for the first time that Shp1 selectively participates in α4β1 but not αLβ2 integrin activation in PC, possibly reflecting the more dominant role of α4β1 over αLβ2 in mediating the homing of cells to the bone marrow [55] . Integrins are essential for ASC to egress from secondary lymphoid organs [25] . It is known that integrin-mediated cell contacts are transient and perturbations of the kinetics of integrin-mediated cell adhesion and de-adhesion might affect cell migration [44] , [45] , [54] , [56] . Neutrophils from motheaten and motheaten viable mice are hyperadhesive and could not de-adhere due to exaggerated integrin signalling [57] . We also hypothesize that in the absence of Shp1, α4β1 integrins were aberrantly activated and failed to detach from its cognate ligand in the spleen and therefore affected PC homing to the bone marrow. In support of this hypothesis, we demonstrated that LPS-activated Shp1-deficient B cells showed reduced movement on VCAM-1-coated surfaces. LPS-differentiated mutant B cells exhibited rounded shapes and were defective in forming polarized morphology like control cells did. Activated mutant PCs were also less efficient in transmigrating across VCAM-1-coated trans-well, resembling the impaired transmigration of cells expressing constitutive active integrin [44] . Histology analysis further revealed that mutant ASC were scattered in the extrafollicular spaces and were unlike wild-type ASC that tend to cluster at the presumably exit sites in the spleen. When equal number of Tat-cre-transduced, LPS-stimulated Ptpn6 +/+ and Ptpn6 f/f cells were reconstituted in vivo , Shp1-deficient PCs could not home to the bone marrow. Finally, when α4β1–VCAM-1 interaction was blocked in immunized Ptpn6 f/f Aicda Cre/+ mice, we were able to detect increased ASC in the bone marrow. Thus, the impaired migration of newly generated splenic Shp1-deficient ASC to their destined niche in the bone marrow as a result of enhanced α4β1 activation might account for the reduced long-lived PC pool and defective humoral immune response in Ptpn6 f/f Aicda Cre/+ mice. To elucidate the mechanism of how Shp1-deficiency affects integrin activation, we investigated signalling pathways downstream of integrin activation. Shp1 is known to dephosphorylate Src family kinase member Lyn (refs 11 , 58 , 59 ), which has been shown to be important for integrin function [60] , [61] . PI3-kinase and AKT were also reported to be aberrantly activated in motheaten mice [10] , and PI3-kinase/AKT signalling cascade is essential for integrin outside-in signalling [62] . Constitutive AKT signalling is known to inhibit the homing of haematopoietic progenitors [63] . We detected increased Src- and PI3-kinase and AKT activation in Shp1-deficient plasmablasts that exhibited enhanced α4β1 integrin-binding activity. Integrin-binding affinity of Shp1-deficient plasmablasts could be restored to normalcy when Src family kinase and PI3-kinase inhibitors were added, indicating that the hyperactivation of these signalling pathways in the absence of Shp1 leads to aberrant integrin activation. The binding of wild-type plasmablasts to VCAM-1 was also affected when Src family kinase and PI3-kinase inhibitors were added, which is consistent with reported roles of Src family kinase and PI3-kinase in integrin activation in other cell types [64] . In summary, we have deleted Shp1 specifically in activated B cells and this leads to hyperactivation of Src family kinase and PI3-kinase signalling and manifests exaggerated α4β1 binding affinity. Both kinases are important in mediating cell migration [48] , and dysregulation of these kinases might be responsible for the PC defects seen in Ptpn6 f/f Aicda Cre/+ mice. Dysregulated integrin signalling deters PCs from migrating from the site of generation to the long-lived niche in the bone marrow. Mouse immunization and antibody treatment Ptpn6 f/f mice were obtained from the Jackson Laboratory. Aicda Cre /+ mice were generated in the laboratory of Nancy Jenkins by knocking in Cre cDNA between the stop codon and 3′-untranslated region of Aicda [65] . Ptpn6 f/f mice were bred with CD19 Cre/+ or Aicda Cre /+ mice to generate Ptpn6 f/f CD19 Cre/+ or Ptpn6 f/f Aicda Cre /+ mice. Mice were bred and maintained in our animal facilities and used according to guidelines issued by the National Advisory Committee on Laboratory Animal Research. Protocol with IACUC No 110611 was approved by Institutional Animal Care and Use Committee of Agency for Science, Technology and Research (A*STAR), Biological Resource Center (BRC). Steps were taken to minimize animal suffering. Floxed (550 bp) and deleted (330 bp) Ptpn6 alleles were identified by PCR [17] . Sex-matched 8–12-week-old mice were immunized with 100 μg NP 38 -chicken γ-globulin (CGG; Biosearch Technologies) in Imject alum (Pierce Biotechnology) by intraperitoneal injection. NP 38 -chicken γ-globulin (100 μg) in PBS was used for secondary immunization where applicable. For VCAM-1 blocking study, mice were i.v. injected with anti-VCAM-1 mAb (Clone 429 MVCAM.A, rat IgG2a, 100 μg per mouse; BD Biosciences) at 10 days after antigenic challenge. Control mice were given purified isotype-matched, irrelevant IgG2a mAb (R35-95, 100 μg per mouse; BD Biosciences). Flow cytometry and cell sorting Single-cell suspensions from spleens, BM, peritoneal cavity (PerC), inguinal lymph nodes (LN) and PP were prepared and stained with various combinations of fluorochrome-conjugated antibodies to CD19, CD38, β1, αLβ2, CXCR4, CD138, B220 (BioLegend), IgM, IgD, CD5, CD43, CD23, Fas (BD Biosciences). 4′,6-diamidino-2-phenylindole (Sigma-Aldrich) were used to exclude dead cells. Antigen-specific B cells were detected with anti-B220, Dump, anti-IgG1 antibodies and NIP. PE-labelled NIP-BSA (Biosearch Technologies) was prepared using APC or R-PE labelling kit-SH (Dojindo). Exclusion staining (Dump) of cells included anti-IgD, anti-CD138, anti-CD3, anti-Th1.2, anti–Gr-1, anti-F4/80, anti-Ter119, anti-DX5, anti-NK1.1, anti-AA4.1 and anti-CD5 mAbs. Antibodies were diluted (1:100) in PBS containing 5% fetal bovine serum. Samples were acquired on an LSR II cytometer (BD Biosciences) and analysed with FlowJo software (TreeStar). For intracellular staining of Shp1, PP GC B cells were stained with PE-anti-Shp1 (Santa Cruz), using BD Cytofix/Cytoperm Kit (BD Biosciences), following manufacturer’s instructions. The expression of phospho-AKT, phospho-Syk (Cell Signaling) and phospho-ERK 1/2 (BD Biosciences) in LPS-differentiated plasmablast were measured by flow cytometry using BD Phosflow kit for mouse splenocytes (BD Biosciences). Briefly, cells were directly fixed in Phosflow Buffer I for 10 min at 37 °C. After washing, permeabilization was performed with Phosflow Perm Buffer I for 30 min at room temperature. Then, cells were washed twice and stained for 30 min at room temperature in dark with anti-phospho-AKT, anti-phospho-Syk, anti-phospho-ERK, anti-CD138 and anti-B220. For cell isolation, CD19 + CD38 − Fas + activated B cells and CD19 + CD38 + Fas − non-activated B cells from the PPs of unimmunized mice, and LPS-differentiated B220 low CD138 + plasmablast were sorted with FACSAria (BD Biosciences). ELISA and ELISPOT NP-specific IgM and IgG1 antibodies and ASCs were detected via ELISA and ELISPOT, respectively. Briefly, 386-well flat-bottom plates (NUNC) were coated with 5 μg ml −1 of NP 14 -BSA or NP 2 -BSA and blocked with 2% BSA in PBS. Serially diluted sera were added. After washing, the plates were incubated with biotinylated anti-IgM and anti-IgG1 antibodies (diluted 1:1,000 in 2% BSA in PBS) followed by streptavidin-conjugated HRP. Bound secondary antibodies were assessed by incubation with 3,3′,5,5′ tetramethyl benzidine thiobarbituric acid substrate. To analyse the frequency of antibody-forming cells, ELISPOT assay was performed using MultiScreen filter plates (Millipore). B-cell isolation and TAT-Cre transduction B cells were isolated from the spleens of Ptpn6 +/+ and Ptpn6 f/f mice by negative selection using CD43 microbeads (Miltenyi Biotec). After three washes with HyQADCF-Mab medium (Hyclone), 1 × 10 7 cells per ml were incubated for 45 min at 37 °C with TAT-Cre at a concentration of 35 mg ml −1 (ref. 66 ). Cells were again washed twice with RPMI medium plus 10% FBS, and cultured for 3 days at a density of 2 × 10 6 cells per ml with LPS (20 μg ml −1 ) to induce plasmablast in vitro . In vivo bone marrow homing of labelled cells TAT-Cre-transduced and LPS-differentiated Ptpn6 +/+ or Ptpn6 f/f cells were incubated with 0.2 mM CellTracker (CT) Green 5-chloromethylfluorescein diacetate (CMFDA; Molecular Probes) or 5 mM CT Orange 5-chloromethyl tetramethylrhodamine, respectively, at 37 °C for 45 min. The two cell preparations were washed and counted, then mixed together to achieve 1:1 ratio for i.v. injection into recipient 8–12-week-old C57BL/6 mice for a period of 16 h. A correction factor was applied to the subsequent data if the lymphocyte ratio was not precisely 1:1. In general, a total of 2 × 10 7 cells in a volume of 200 μl was injected per tail vein. Recovered Ptpn6 +/+ and Ptpn6 f/f PC numbers were normalized to per cent of PCs. Soluble ligand-binding assay Splenocytes from immunized mice or LPS-differentiated cells (2 × 10 6 per 100 μl of RPMI containing 1 mM MgCl 2 and 1 mMCaCl 2 ) were incubated with soluble ICAM-1/VCAM-1 conjugated to human Fc (20 μg ml −1 ; R&D Systems) for 30 min at room temperature, with or without inhibitors to Src family tyrosine kinases (PP2,10 μM) or PI3-kinase (LY294002,10 μM). Binding of ICAM-1/VCAM-1 was detected by incubating cells with APC-conjugated anti-human Fc (BioLegend) for 20 min at 4 °C, followed by dual staining with anti-CD138 and anti-B220 for 20 min at 4 °C to identify ASCs by flow cytometry. Antibodies were diluted (1:100) in PBS containing 5% fetal bovine serum. Transmigration assays For transmigration assays, the upper chamber of the trans-well was non-coated or coated with VCAM-1 (40 μg/ml) for 2 h at 37 °C. A total of 10 6 sorted plasmablasts were added to the upper chamber and allowed to transmigrate for 4 h to the lower chamber that contained 2 μg ml −1 CXCL12 (SDF-1α) at 37 °C and 5% CO 2 . Migrated cells were counted in a LSR II flow cytometer by passing each sample in the same predetermined time and flow conditions. Migrated cells were represented as the percentage of total cell input. Assays were performed in triplicate. Histology Spleens sections were harvested, embedded in Tissue-Tek and ‘snap-frozen’ in dry ice and stored at −80 °C. Cryostat sections (8 μm in thickness) were prepared, air-dried and fixed in ice-cold acetone for 15 min. Sections were blocked with 5% rat serum and stained with the following antibodies: anti-IgG1, anti-IgD, anti-CD3 or anti-VCAM-1 antibodies (BD Biosciences PharMingen). Antibodies were diluted (1:50) in PBS containing 5% rat serum. Sections were further mounted with CYTOSEAL 60 (Electron Microscopy Sciences) and analysed with an Olympus FV1000 microscope (Olympus) using a × 20 objective, and the images were acquired with Olympus Fluoview Version 2.1 software. Videomicroscopy A glass-bottomed 35-mm dish was coated with VCAM-1 (20 μg ml −1 ) at 4 °C overnight. Cells were allowed to adhere to the VCAM-1-coated dish for 15 min at 37 °C. The dish containing cells was mounted with an adaptor onto the stage of Olympus microscope with a closed humidified system with temperature (37 °C) and CO 2 control. Images of live cells were acquired with Olympus Fluoview Version 2.1 software using × 20 objectives at an interval of 1 min and analysed using the softwares xcellence rt (Olympus) and Imaris (Bitplane scientific software). Immunoblot analysis Whole-cell lysates of sorted non-plasmablast or plasmablast were separated by SDS–PAGE and blotted using standard procedures. The following antibodies were used: phospho-Shp1 (Tyr564), phospho-Src family kinase (Tyr416) (Cell Signaling), phospho-PI3-kinase p85α (Santa Cruz), c-Src (Cell Signaling) and PI3-kinase p85α (Upstate). The membranes were incubated with horseradish peroxidase-conjugated secondary antibodies (Santa Cruz), and visualized with SuperSignal West Pico/Dura chemiluminescent substrate (Pierce). qRT-PCR analyses Total RNA was isolated using isopropanol precipitation, and the cDNA was prepared with the RevertAid H Minus First-Strand cDNA Synthesis Kit (Fermentas). SYBR Green Master Mix (Applied Biosystems) was used for real-time PCR on an ABI Prism7500 instrument (Applied Biosystems). The mRNA level was normalized to the expression of β-actin mRNA. The primer sequences were as follows: SHP1 forward, 5′-CTTGGCAGGAGAACACTCGT-3′, SHP1 reverse, 5′-ACCATAGACACGCTGAGTGC-3′; β-actin forward, 5′-AGGCACCAGGGCGTGAT-3′, β-actin reverse, 5′-GCCCACATAGGAATCCTTCTGAC-3′. Statistics Two-tailed Student’s t -test was used for statistical analyses. How to cite this article: Li, Y.-F. et al . Shp1 signalling is required to establish the long-lived bone marrow plasma cell pool. Nat. Commun. 5:4273 doi: 10.1038/ncomms5273 (2014).